Ongoing activation of sphingosine 1-phosphate receptors mediates maturation of exosomal multivesicular endosomes During late endosome maturation, cargo molecules are sorted into intralumenal vesicles (ILVs) of multivesicular endosomes (MVEs), and are either delivered to lysosomes for degradation or fused with the plasma membranes for exosome release. The mechanism underlying formation of exosomal ILVs and cargo sorting into ILVs destined for exosome release is still unclear. Here we show that inhibitory G protein (Gi)-coupled sphingosine 1-phosphate (S1P) receptors regulate exosomal MVE maturation. Gi-coupled S1P receptors on MVEs are constitutively activated through a constant supply of S1P via autocrine activation within organelles. We also found that the continuous activation of Gi-coupled S1P receptors on MVEs is essential for cargo sorting into ILVs destined for exosome release. Our results reveal a mechanism underlying ESCRT-independent maturation of exosomal MVEs. Endocytosis is a fundamental property of eukaryotic cells and is the means by which cell membrane proteins and solutes are internalized and delivered to endosomal compartments. During endosomal maturation, cargo molecules are sorted into intralumenal vesicles (ILVs) of multivesicular endosomes (MVEs), and are then delivered to lysosomes for degradation [1] , [2] . It is well known that cargo molecules such as epidermal growth factor (EGF) receptor are ubiquitinated and sorted into ILVs, which is destined for lysosomal degradation, in an endosomal-sorting complex required for transport (ESCRT) machinery-dependent manner [3] , [4] , [5] , [6] , [7] , [8] , [9] , [10] , [11] , [12] , [13] , [14] , [15] , [16] . In this system, a phospholipid metabolite, lysobisphoshatidic acid, has also been shown to have a role in ILV formation [17] . Alternatively, MVEs can directly fuse with the plasma membranes, leading to release of the ILVs into the extracellular environment as exosomes [18] , [19] . Exosomes are small membrane-bound vesicles with a diameter of 50–100 nm released from a variety of cells important for erythrocyte maturation, cell-to-cell communication, antigen presentation, prion diseases, tumour metastasis and Alzheimer’s disease [20] , [21] , [22] , [23] , [24] , [25] . Recently, it has been reported that CD63, which is enriched in exosomes, is sorted into ILVs by an ESCRT machinery-independent manner [26] . Likewise, the melanosomal protein Pmel17 in melanoma cells [27] and major histocompatibility complex class II molecules in activated dendritic cells [28] are inserted into ILVs independently of ubiquitination. In addition, the CD63 itself is required for normal Pmel to be sorted into luminal domain in an ESCRT-independent manner [29] . A factor involved in ESCRT-independent ILV biogenesis has recently been proposed, that is, a sphingolipid metabolite ceramide, which have been demonstrated to spontaneously induce formation of internal vesicles in liposomes in vitro [30] . They also showed that secreted exosomes contain high concentrations of ceramide. However, the precise mechanisms underlying cargo sorting into exosomal ILVs are still unknown. As for ceramide formation, sphingomyelin at the membrane raft undergoes enzymatic cleavage to ceramide and phosphorylcholine by various sphingomyelinases. Once the sphingomyelin cycle is initiated, ceramide is subject to a number of metabolic fates, including its catabolism to sphingosine and sphingosine 1-phosphate (S1P), and these lipid metabolites elicit diverse cellular functions as lipid mediators [31] . It is well known that the S1P acts as an extracellular ligand, which binds to S1P receptors on the plasma membranes and regulates a variety of cell functions [32] , [33] . All S1P receptors (type 1–5) are classified into a family of G protein-coupled receptors and show distinct expression in tissues and cells, and also show unique G protein-coupling patterns, suggesting distinctive functions [34] . We reasoned that S1P signalling might be involved in the exosomal MVE maturation, because the subunits of G proteins are known to be involved in various types of fission/fusion events in vesicular trafficking [35] , [36] , [37] and protein sorting [38] . In the present studies, we have found that inhibitory G protein (Gi)-coupled S1P receptors on MVEs undergo continuous activation through a constant supply of S1P within the organelles. Functional studies have revealed that S1P signalling is critical in the cargo sorting into exosomal ILVs. The importance of sphingolipid metabolites in the formation of and cargo sorting into exosomal ILVs are discussed herein. Gi-coupled receptors are continuously activated on MVEs To detect the activation state of endogenous Gi-coupled receptors, fluorescence resonance energy transfer (FRET) analysis using Gi subunit pairs was employed ( Fig. 1a ). The α-subunit of Gi (Gαi)-cyan fluorescent protein (CFP) and the γ-subunit of G protein (Gγ)-yellow fluorescent protein (YFP) [39] were expressed in HeLa cells, and after fixation Gi-coupled receptor activation at various cellular sites was assessed by FRET analysis using acceptor photobleaching. After Gγ-YFP at the plasma membrane areas was photobleached, Gαi-CFP signal was augmented ( Fig. 1b,c , green squared area, and Supplementary Fig. S1 ), indicating elevated FRET efficiency, an associated form of the Gi protein (non-activated state, Fig. 1a ). FRET efficiency at plasma membranes decreased (activated state) on stimulation by the addition of agonist, ADP or S1P, which is known to bind to the Gi-coupled P2Y or S1P receptor, respectively ( Fig. 1d,e and Supplementary Figs S1 and S2 ), confirming that each Gi-coupled receptor activation at the plasma membranes causes a transient dissociation of Gi subunits, that is, being rapidly activated (dissociated) on agonist stimulation and returned to the non-activated state (re-associated) within 20 min. Unexpectedly, the FRET efficiency at cellular vesicles was consistently low ( Fig. 1b,c , red circled area, and Supplementary Fig. S1 ), indicating an activated (dissociated) state of the Gi protein under basal conditions. It is noteworthy that treatment of the cells with pertussis toxin (PTX), which is known to make Gi-coupled receptors refractory to agonists [40] , resulted in an enhanced FRET efficiency at the cellular vesicles as well as at the plasma membranes ( Fig. 1f and Supplementary Figs S1 and S2 ). These results strongly suggest that the Gi-coupled receptors at the cellular vesicles are being continuously activated in situ . The Gi-associated vesicles were further characterized by their localization patterns with authentic vesicle markers. Among various marker proteins tested, the Gi-positive vesicles co-localized well with a late endosome/MVE marker, CD63, whereas they did not co-localize with an early endosome marker, early endosome antigen 1 (EEA1; Fig. 1g ). 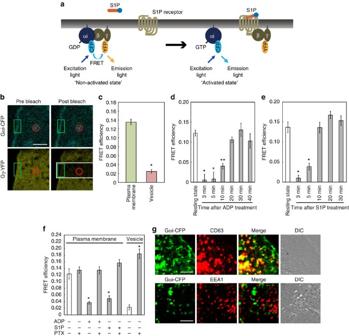Figure 1: Ongoing activation of Gi-coupled receptors on CD63-positive vesicles. (a) The strategy to detect endogenous Gi-coupled receptor activation using FRET is depicted. The FRET probes, Gαi-CFP and Gγ-YFP were prepared. When these constructs are excited with CFP excitation light, emission light is shifted from cyan to yellow when both fluorophores are close enough to each other under ‘non-activated state’ to permit FRET. (b) HeLa cells transiently expressing Gαi-CFP, Gβ and Gγ-YFP were fixed, and YFP at a selected area (white square) was photobleached. The fluorescence intensity of CFP at the plasma membranes (green squares) and the vesicles (red circles) before and after photobleaching was analysed by confocal microscopy. Scale bar, 5 μm. (c) The FRET efficiency was calculated from the results inb. Values represent means±s.e.m. (n≥90 endosomes; *P<0.001; Welch’st-test). (d) HeLa cells expressing Gαi-CFP, Gβ and Gγ-YFP were incubated with 100 μM ADP at 4 °C for 1 h. After washing out, the medium cells were replaced with fresh medium, incubated for the indicated time at 37 °C and fixed. The FRET efficiency at plasma membrane areas was measured by confocal microscopy. Values represent means±s.e.m. (n≥41 endosomes; *P<0.001, **P<0.005 versus resting state (open); Welch’st-test). (e) HeLa cells expressing Gαi-CFP, Gβ and Gγ-YFP were incubated with 100 nM S1P at 4 °C for 1 h. After washing out, the medium cells were replaced with fresh medium, incubated for the indicated time at 37 °C, fixed and followed by FRET analysis as ind. Values represent means±s.e.m. (n≥59 endosomes; *P<0.001 versus resting state (open); Welch’st-test). (f) HeLa cells expressing Gαi-CFP, Gβ and Gγ-YFP were pretreated with or without 100 ng ml−1PTX for 24 h, stimulated with or without 100 μM ADP or 100 nM S1P for 5 min and fixed. The FRET efficiency at the specified areas was measured. Values represent means±s.e.m. (n≥32; *P<0.001 versus treatment free (open); Welch’st-test). (g) HeLa cells expressing Gαi-CFP were immunostained with anti-CD63 or anti-EEA1 antibodies. Scale bar, 5 μm. Figure 1: Ongoing activation of Gi-coupled receptors on CD63-positive vesicles. ( a ) The strategy to detect endogenous Gi-coupled receptor activation using FRET is depicted. The FRET probes, Gαi-CFP and Gγ-YFP were prepared. When these constructs are excited with CFP excitation light, emission light is shifted from cyan to yellow when both fluorophores are close enough to each other under ‘non-activated state’ to permit FRET. ( b ) HeLa cells transiently expressing Gαi-CFP, Gβ and Gγ-YFP were fixed, and YFP at a selected area (white square) was photobleached. The fluorescence intensity of CFP at the plasma membranes (green squares) and the vesicles (red circles) before and after photobleaching was analysed by confocal microscopy. Scale bar, 5 μm. ( c ) The FRET efficiency was calculated from the results in b . Values represent means±s.e.m. ( n ≥90 endosomes; * P <0.001; Welch’s t -test). ( d ) HeLa cells expressing Gαi-CFP, Gβ and Gγ-YFP were incubated with 100 μM ADP at 4 °C for 1 h. After washing out, the medium cells were replaced with fresh medium, incubated for the indicated time at 37 °C and fixed. The FRET efficiency at plasma membrane areas was measured by confocal microscopy. Values represent means±s.e.m. ( n ≥41 endosomes; * P <0.001, ** P <0.005 versus resting state (open); Welch’s t -test). ( e ) HeLa cells expressing Gαi-CFP, Gβ and Gγ-YFP were incubated with 100 nM S1P at 4 °C for 1 h. After washing out, the medium cells were replaced with fresh medium, incubated for the indicated time at 37 °C, fixed and followed by FRET analysis as in d . Values represent means±s.e.m. ( n ≥59 endosomes; * P <0.001 versus resting state (open); Welch’s t -test). ( f ) HeLa cells expressing Gαi-CFP, Gβ and Gγ-YFP were pretreated with or without 100 ng ml −1 PTX for 24 h, stimulated with or without 100 μM ADP or 100 nM S1P for 5 min and fixed. The FRET efficiency at the specified areas was measured. Values represent means±s.e.m. ( n ≥32; * P <0.001 versus treatment free (open); Welch’s t -test). ( g ) HeLa cells expressing Gαi-CFP were immunostained with anti-CD63 or anti-EEA1 antibodies. Scale bar, 5 μm. Full size image S1P receptors are continuously activated on MVEs We next tried to identify the Gi-coupled receptors on the CD63-positive MVEs. Our previous observation that PTX-sensitive S1P receptors were involved in vesicular trafficking and involved in glutamate release from internal vesicles in hippocampal neurons [41] prompted us to ask whether S1P receptors may be involved in the ‘ongoing activation’ of Gi-coupled receptors on the CD63-positive MVEs. To address this possibility, functional involvement of S1P receptors on these MVEs was assessed by FRET analysis using the Gi subunit pair in each S1P receptor subtype-depleted cells. Importantly, FRET efficiency using Gαi/Gγ pair largely increased (associated, non-activated state) in S1P 1 or S1P 3 receptor-short interfering RNA (siRNA)-treated but not in S1P 2 receptor-siRNA-treated cells as compared with that treated with control siRNA ( Fig. 2a and Supplementary Figs S1 and S2 ), suggesting the involvement of S1P 1 and/or S1P 3 receptors in these phenomena. Indeed, an S1P 1 antagonist, W146, strongly, and an S1P 3 antagonist, BML-241, moderately, but not an S1P 2 antagonist, JTE-013, increased the FRET efficiency ( Fig. 2b and Supplementary Figs S1 and S2 ). Furthermore, transiently expressed S1P 1 -YFP or green fluorescent protein (GFP)-tagged S1P 3 (S1P 3 -GFP) but not S1P 2 -GFP showed a good co-localization with CD63-mCherry ( Supplementary Figs S3 and S6c ). Taken together, S1P 1 and/or S1P 3 receptors may be continuously activated on CD63-positive MVEs. 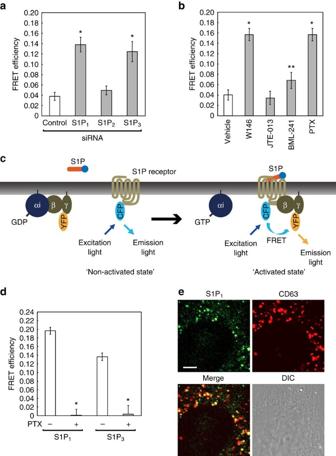Figure 2: Identification of Gi-coupled receptors continuously activated on CD63-positive MVEs as S1P1/S1P3receptors. (a) HeLa cells cotransfected with either control, hS1P1-, hS1P2- or hS1P3-siRNA, together with vectors encoding Gαi-CFP, Gβ, Gγ-YFP and CD63-mCherry were fixed. The FRET efficiency was measured at CD63-mCherry-positive vesicle areas. Values represent means±s.e.m. (n≥34; *P<0.001 versus control siRNA (open); Welch’st-test). (b) HeLa cells expressing Gαi-CFP, Gβ, Gγ-YFP and CD63-mCherry were treated with or without 10 μM W146, 5 μM JTE-013, 10 μM BML-241 or 100 ng ml−1PTX for 24 h, fixed and followed by FRET analysis as ina. Values represent means±s.e.m. (n≥34; *P<0.001, **P<0.05 versus vehicle (open); Welch’st-test). (c) The strategy to detect S1P receptor activation using FRET is depicted. The FRET probes, S1P receptor subtype-CFP and Gγ-YFP were prepared. When these constructs are excited with CFP excitation light, emission light is shifted from cyan to yellow when both fluorophores are close enough to each other under ‘activated state’ to permit FRET. (d) HeLa cells expressing S1P1-CFP, Gβ, Gγ-YFP and CD63-mCherry or S1P3-CFP, Gβ, Gγ-YFP and CD63-mCherry were treated with or without 100 ng ml−1PTX for 24 h, fixed and followed by FRET analysis as ina. Values represent means±s.e.m. (n≥51; *P<0.001 versus PTX-free (open); Welch’st-test). (e) HeLa cells were immunostained for endogenous S1P1and CD63 with respective antibodies. Scale bar, 5 μm. Figure 2: Identification of Gi-coupled receptors continuously activated on CD63-positive MVEs as S1P 1 /S1P 3 receptors. ( a ) HeLa cells cotransfected with either control, hS1P 1 -, hS1P 2 - or hS1P 3 -siRNA, together with vectors encoding Gαi-CFP, Gβ, Gγ-YFP and CD63-mCherry were fixed. The FRET efficiency was measured at CD63-mCherry-positive vesicle areas. Values represent means±s.e.m. ( n ≥34; * P <0.001 versus control siRNA (open); Welch’s t -test). ( b ) HeLa cells expressing Gαi-CFP, Gβ, Gγ-YFP and CD63-mCherry were treated with or without 10 μM W146, 5 μM JTE-013, 10 μM BML-241 or 100 ng ml −1 PTX for 24 h, fixed and followed by FRET analysis as in a . Values represent means±s.e.m. ( n ≥34; * P <0.001, ** P <0.05 versus vehicle (open); Welch’s t -test). ( c ) The strategy to detect S1P receptor activation using FRET is depicted. The FRET probes, S1P receptor subtype-CFP and Gγ-YFP were prepared. When these constructs are excited with CFP excitation light, emission light is shifted from cyan to yellow when both fluorophores are close enough to each other under ‘activated state’ to permit FRET. ( d ) HeLa cells expressing S1P 1 -CFP, Gβ, Gγ-YFP and CD63-mCherry or S1P 3 -CFP, Gβ, Gγ-YFP and CD63-mCherry were treated with or without 100 ng ml −1 PTX for 24 h, fixed and followed by FRET analysis as in a . Values represent means±s.e.m. ( n ≥51; * P <0.001 versus PTX-free (open); Welch’s t -test). ( e ) HeLa cells were immunostained for endogenous S1P 1 and CD63 with respective antibodies. Scale bar, 5 μm. Full size image S1P 1 receptors are known to be coupled exclusively with Gi/o, whereas the S1P 3 receptor is coupled with various G proteins such as Gi/o, Gq or G12/13, depending on cell types [42] . To characterize to what extent Gi is involved in the S1P 3 receptor signal, we conducted a FRET analysis using another FRET pair, that is, an S1P receptor subtype-CFP/Gγ-YFP pair where FRET efficiency increases on receptor stimulation as previously reported [43] ( Fig. 2c and Supplementary Fig. S4 ). To validate further to use the fluorescent protein in the FRET study, we assessed the ability of this protein to internalize on S1P stimulation. The S1P 1 -CFP underwent time-dependent internalization after S1P stimulation ( Supplementary Fig. S5 ) in an agreement with previous reports [44] , [45] . Using this FRET pair, both S1P 1 and S1P 3 receptors were continuously activated on CD63-positive MVEs as judged by FRET analysis using the S1P receptor subtype-CFP/Gγ-YFP pair ( Fig. 2d and Supplementary Figs S1 and S2 ). It should be noted that the FRET efficiency between S1P 3 and Gγ was strongly inhibited by PTX treatment to almost the same extent as with the S1P 1 receptor, indicating S1P 3 receptor is almost exclusively coupled with Gi in HeLa cells. We therefore focused the S1P 1 receptor in the following studies as a representative of Gi-coupled S1P receptors. To begin with, immunocytochemical analysis was performed to detect both endogenous S1P 1 receptor and CD63, showing good co-localization of these proteins on CD63-positive MVEs ( Fig. 2e ). Sphingosine kinase is involved in constant S1P supply on MVEs As a result of the S1P gradient, that is, high S1P concentrations in plasma and low in tissues [46] , we hypothesized that S1P receptors on MVEs may be continuously activated by a constant supply of S1P catalysed by sphingosine kinase (SphK). To prove this, we tested the effect of an SphK inhibitor, 2-(p-hydroxyanilino)-4-(p-chlorophenyl)thiazole (HACPT) on S1P 1 receptor activation as measured by FRET efficiency using an S1P 1 receptor/Gγ pair on MVEs in HeLa cells ( Fig. 3a and Supplementary Figs S1 and S2 ) and primary human umbilical vein endothelial cells (HUVEC; Supplementary Fig. S6a ). Importantly, HACPT treatment caused a decrease (non-activated state) in the FRET efficiency, supporting this hypothesis. To further verify this idea, photolysis-activated caged S1P almost completely rescued the inhibitory effect of HACPT, whereas the non-activated one was inert. Moreover, FRET analysis using a G protein subunit pair ( Fig. 1a ) also confirmed this conclusion ( Fig. 3b and Supplementary Figs S1 and S2 ). 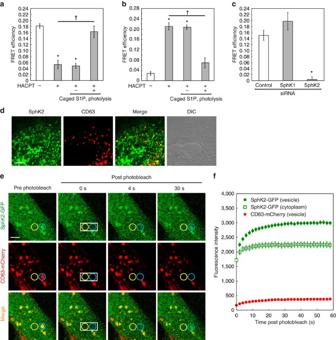Figure 3: Identification of SphK subtypes involved in constant S1P production on CD63-positive MVEs. (a) HeLa cells expressing S1P1-CFP, Gβ, Gγ-YFP and CD63-mCherry were treated with dimethyl sulphoxide vehicle or 5 μM HACPT for 24 h, loaded with 1 μM caged S1P, incubated for another 5 min after photolysis as indicated and fixed. The FRET efficiency was measured at CD63-mCherry-positive vesicle areas. Values represent means±s.e.m. (n≥42; *P<0.001 versus vehicle (open),†P<0.001; Welch’st-test). (b) HeLa cells expressing Gαi-CFP, Gβ, Gγ-YFP and CD63-mCherry were treated with or without 5 μM HACPT for 24 h, loaded with 1 μM caged S1P, incubated for another 5 min after photolysis as indicated, fixed and followed by FRET analysis as ina. Values represent means±s.e.m. (n≥33; *P<0.001 versus vehicle treatment (open),†P<0.001; Welch’st-test). (c) HeLa cells cotransfected with either control, hSphK1- or hSphK2-siRNA together with vectors encoding S1P1-CFP, Gβ, Gγ-YFP and CD63-mCherry were fixed and followed by FRET analysis as ina. Values represent means±s.e.m. (n≥45; *P<0.001 versus control siRNA (open)). (d) HeLa cells were immunostained for endogenous SphK2 and CD63 with respective antibodies. Scale bar, 5 μm. (e) In HeLa cells expressing SphK2-GFP and CD63-mCherry, the area (white squares) including both SphK2-GFP plus CD63-mCherry-positive area (blue circles) and SphK2-GFP alone in adjacent cytoplasmic area (yellow circles) were photobleached. After photobleaching, the recovery of each fluorescence is sequentially shown. Scale bar, 5 μm. (f) A quantified result ofe. Time-dependent recovery of each fluorescence in bleached areas is shown. Values represent means±s.e.m. (n=60). Figure 3: Identification of SphK subtypes involved in constant S1P production on CD63-positive MVEs. ( a ) HeLa cells expressing S1P 1 -CFP, Gβ, Gγ-YFP and CD63-mCherry were treated with dimethyl sulphoxide vehicle or 5 μM HACPT for 24 h, loaded with 1 μM caged S1P, incubated for another 5 min after photolysis as indicated and fixed. The FRET efficiency was measured at CD63-mCherry-positive vesicle areas. Values represent means±s.e.m. ( n ≥42; * P <0.001 versus vehicle (open), † P <0.001; Welch’s t -test). ( b ) HeLa cells expressing Gαi-CFP, Gβ, Gγ-YFP and CD63-mCherry were treated with or without 5 μM HACPT for 24 h, loaded with 1 μM caged S1P, incubated for another 5 min after photolysis as indicated, fixed and followed by FRET analysis as in a . Values represent means±s.e.m. ( n ≥33; * P <0.001 versus vehicle treatment (open), † P <0.001; Welch’s t -test). ( c ) HeLa cells cotransfected with either control, hSphK1- or hSphK2-siRNA together with vectors encoding S1P 1 -CFP, Gβ, Gγ-YFP and CD63-mCherry were fixed and followed by FRET analysis as in a . Values represent means±s.e.m. ( n ≥45; * P <0.001 versus control siRNA (open)). ( d ) HeLa cells were immunostained for endogenous SphK2 and CD63 with respective antibodies. Scale bar, 5 μm. ( e ) In HeLa cells expressing SphK2-GFP and CD63-mCherry, the area (white squares) including both SphK2-GFP plus CD63-mCherry-positive area (blue circles) and SphK2-GFP alone in adjacent cytoplasmic area (yellow circles) were photobleached. After photobleaching, the recovery of each fluorescence is sequentially shown. Scale bar, 5 μm. ( f ) A quantified result of e . Time-dependent recovery of each fluorescence in bleached areas is shown. Values represent means±s.e.m. ( n =60). Full size image Next, we sought to determine SphK subtypes responsible for the production of S1P on CD63-positive MVEs. FRET efficiency using an S1P 1 receptor/Gγ pair ( Fig. 2c ) was measured in each SphK subtype-depleted cells. SphK1-siRNA treatment showed almost no significant changes compared with the control siRNA-treated HeLa cells ( Fig. 3c and Supplementary Figs S1 and S2 ) or HUVEC ( Supplementary Fig. S6b ). However, SphK2-siRNA treatment caused robust inhibition of the FRET efficiency (non-activated state), suggesting SphK2 is responsible for the production of S1P on these MVEs. Indeed, under conditions in which cytoplasmic SphK2 level decreases by serum starvation, the FRET efficiency also decreases ( Supplementary Fig. S7 and see Discussion). FRET analysis using a G protein subunit pair ( Fig. 1a ) also confirmed the involvement of SphK2 in this phenomenon ( Supplementary Fig. S8a ). To support these observations, transiently expressed SphK2-GFP showed a good co-localization with CD63-mCherry, whereas SphK1-GFP did not ( Supplementary Figs S6c and S8b ). Indeed, endogenous SphK2 and CD63 were well co-localized as assessed by immunocytochemistry ( Fig. 3d ). Taken together, the phenomena of SphK2-mediated constant supply of S1P and activation of S1P receptor on MVEs are not restricted to HeLa cells, a cancer cell line, but are also seen in primary cells such as HUVEC. Next, the dynamics of SphK2 behaviour in the cells was further analysed by fluorescence recovery after photobleaching (FRAP) ( Fig. 3e,f ). After SphK2-GFP on CD63-positive MVEs was photobleached, the fluorescence was rapidly restored to a higher fluorescence level than that of the adjacent cytosolic areas, suggesting that SphK2 is recruited to CD63-positive MVEs with a high affinity. In contrast, the fluorescence of CD63-mCherry, which is an integral membrane protein, remained almost unchanged even more than 1 min after photobleaching. S1P signalling is necessary for exosomal MVE maturation The effects of S1P signalling on MVE maturation were studied next. CD63-GFP was transiently expressed in HeLa cells, where the S1P 1 receptor, SphK2 or hepatocyte growth factor-regulated tyrosine kinase substrate (Hrs) was depleted by each molecule-specific siRNA. After treatment of cells with Alexa647-EGF, CD63 or EGF fluorescence in MVEs was measured. Intriguingly, depletion of S1P 1 receptor expression caused a significant decrease in CD63 intensity in EGF-negative exosomal MVEs as compared with that in control siRNA-treated cells ( Fig. 4a,b ). In addition, depletion of SphK2, which is required for the continuous activation of the S1P 1 receptors on CD63-positive MVEs ( Fig and Supplementary Fig. S8a ), caused a decrease in CD63 intensity in EGF-negative exosomal MVEs. On the other hand, depletion of Hrs, which is known to be required for ESCRT-dependent cargo sorting into ILVs [8] , [11] , [16] , [47] , had almost no effect on CD63 sorting in EGF-negative exosomal MVEs. It is a sharp contrast that depletion of Hrs caused a strong inhibition of EGF sorting into ILVs in EGF-positive MVEs ( Fig. 4a,c ), which is well known as a marker of degradation pathway and to utilize ESCRT machinery. These results imply that the mechanism underlying CD63 sorting into exosomal ILVs is ESCRT-independent, but under the control of S1P signalling. To strengthen this idea, the sorting of cargo molecules such as CD81 and flotillin, known for exosome markers, are all under the control of S1P signalling molecules, S1P 1 receptor and SphK2 ( Fig. 4d,e ). Furthermore, treatment of cells with FTY720, an S1P receptor modulator, caused a strong decrease in the amount of CD63 as well as S1P 1 receptor in exosomal MVEs ( Supplementary Fig. S9 and see Discussion). 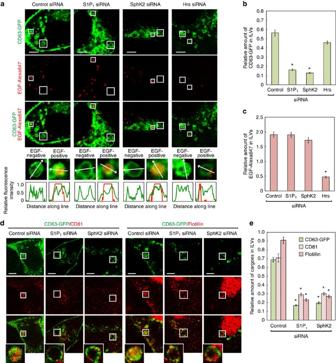Figure 4: Critical role of S1P signalling in exosomal MVE maturation. (a) HeLa cells cotransfected with control, hS1P1-, hSphK2- or hHrs-siRNA together with vectors encoding CD63-GFP and Rab5 (Q79L)-DsRed were incubated with 100 ng ml−1Alexa647-EGF for 30 min and fixed. The fluorescence intensity corresponding to CD63-GFP (green) and Alexa647-EGF (red) within the EGF-negative or -positive enlarged MVEs (boxed) were analysed by line intensity profiles across the cell. Scale bars, 5 μm. (b) Fluorescence intensity of the CD63-GFP sorted in ILVs as inawas quantified. Values represent means±s.e.m. (n≥94; *P<0.001 versus control siRNA; Welch’st-test). (c) Fluorescence intensity of the Alexa647-EGF sorted in ILVs as inawas quantified. Values represent means±s.e.m. (n≥46; *P<0.001 versus control siRNA; Welch’st-test). (d) HeLa cells cotransfected with control, hS1P1- or hSphK2-siRNA together with vectors encoding CD63-GFP and FLAG-Rab5 (Q79L) were fixed, immunostained with anti-CD81 or anti-flotillin antibody. Enlarged MVEs (boxed areas) were analysed by confocal microscopy. Scale bars, 5 μm. (e) Each fluorescence intensity corresponding to CD63-GFP, CD81 and flotillin sorted to ILVs as indwere quantified. Values represent means±s.e.m. (n≥40; *P<0.001 versus control siRNA; Welch’st-test). Figure 4: Critical role of S1P signalling in exosomal MVE maturation. ( a ) HeLa cells cotransfected with control, hS1P 1 -, hSphK2- or hHrs-siRNA together with vectors encoding CD63-GFP and Rab5 (Q79L)-DsRed were incubated with 100 ng ml −1 Alexa647-EGF for 30 min and fixed. The fluorescence intensity corresponding to CD63-GFP (green) and Alexa647-EGF (red) within the EGF-negative or -positive enlarged MVEs (boxed) were analysed by line intensity profiles across the cell. Scale bars, 5 μm. ( b ) Fluorescence intensity of the CD63-GFP sorted in ILVs as in a was quantified. Values represent means±s.e.m. ( n ≥94; * P <0.001 versus control siRNA; Welch’s t -test). ( c ) Fluorescence intensity of the Alexa647-EGF sorted in ILVs as in a was quantified. Values represent means±s.e.m. ( n ≥46; * P <0.001 versus control siRNA; Welch’s t -test). ( d ) HeLa cells cotransfected with control, hS1P 1 - or hSphK2-siRNA together with vectors encoding CD63-GFP and FLAG-Rab5 (Q79L) were fixed, immunostained with anti-CD81 or anti-flotillin antibody. Enlarged MVEs (boxed areas) were analysed by confocal microscopy. Scale bars, 5 μm. ( e ) Each fluorescence intensity corresponding to CD63-GFP, CD81 and flotillin sorted to ILVs as in d were quantified. Values represent means±s.e.m. ( n ≥40; * P <0.001 versus control siRNA; Welch’s t -test). Full size image S1P signalling regulates exosomal cargo sorting into ILVs Next, the dynamics of CD63 sorting into exosomal ILVs were analysed using the FRAP technique. Under control vehicle conditions, fluorescence corresponding to CD63 in exosomal ILVs recovered almost completely within 5 min after photobleaching, indicating active ongoing sorting of this protein ( Fig. 5a,b , upper panels, and Supplementary Movie 1 ). However, the fluorescence intensity remained almost unchanged during the first 5 min after photobleaching in the HACPT-treated cells ( Fig. 5a,b , middle panels, and Supplementary Movie 1 ). This inhibition of CD63 sorting into exosomal ILVs was cancelled by a photolysis-activated caged S1P, confirming the importance of S1P signalling in cargo sorting into exosomal ILVs. Importantly, the S1P action on CD63 sorting was abolished in PTX-treated cells and not rescued by the photolysis-activated caged S1P, indicating that this lipid mediator acts in a receptor-mediated fashion ( Fig. 5a,b , bottom panels). 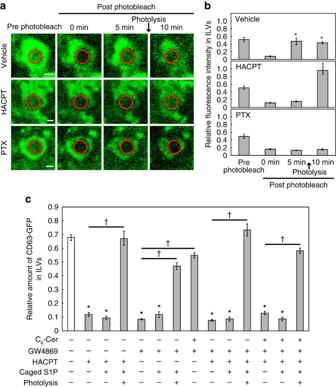Figure 5: Regulation of exosomal cargo sorting into ILVs by receptor-mediated S1P signalling. (a) HeLa cells expressing CD63-GFP and Rab5 (Q79L)-DsRed were pretreated with dimethyl sulphoxide (DMSO) vehicle, 5 μM HACPT or 100 ng ml−1PTX, and 1 μM caged S1P. The areas of endosomal lumen including CD63-GFP-positive enlarged MVEs (red circles) were photobleached and then the fluorescence recovery was sequentially monitored by confocal microscopy. Scale bars, 1 μm. (b) The fluorescence intensity corresponding to CD63-GFP sorted to the ILVs as inawas quantified. Values represent means±s.e.m. (n≥14 endosomes; *P<0.001 versus 0 min of post-photobleach; Welch’st-test). (c) HeLa cells expressing CD63-GFP and Rab5 (Q79L)-DsRed were pretreated with DMSO vehicle or 5 μM neutral sphingomyelinase inhibitor GW4869 for 24 h then pretreated with 5 μM HACPT for 30 min and/or loaded with 1 μM caged S1P for 30 min followed by the treatment with 10 μM C6-ceramide for 6 h as indicated. In some experiments, cells were subjected to ultraviolet radiation leading to photolysis and activation of caged S1P. Cells were fixed and analysed for fluorescence intensity corresponding to the areas where CD63-GFP was sorted to ILVs in enlarged MVEs. Values represent means±s.e.m. (n≥48 endosomes; *P<0.001 versus vehicle (open),†P<0.001; Welch’st-test). Figure 5: Regulation of exosomal cargo sorting into ILVs by receptor-mediated S1P signalling. ( a ) HeLa cells expressing CD63-GFP and Rab5 (Q79L)-DsRed were pretreated with dimethyl sulphoxide (DMSO) vehicle, 5 μM HACPT or 100 ng ml −1 PTX, and 1 μM caged S1P. The areas of endosomal lumen including CD63-GFP-positive enlarged MVEs (red circles) were photobleached and then the fluorescence recovery was sequentially monitored by confocal microscopy. Scale bars, 1 μm. ( b ) The fluorescence intensity corresponding to CD63-GFP sorted to the ILVs as in a was quantified. Values represent means±s.e.m. ( n ≥14 endosomes; * P <0.001 versus 0 min of post-photobleach; Welch’s t -test). ( c ) HeLa cells expressing CD63-GFP and Rab5 (Q79L)-DsRed were pretreated with DMSO vehicle or 5 μM neutral sphingomyelinase inhibitor GW4869 for 24 h then pretreated with 5 μM HACPT for 30 min and/or loaded with 1 μM caged S1P for 30 min followed by the treatment with 10 μM C 6 -ceramide for 6 h as indicated. In some experiments, cells were subjected to ultraviolet radiation leading to photolysis and activation of caged S1P. Cells were fixed and analysed for fluorescence intensity corresponding to the areas where CD63-GFP was sorted to ILVs in enlarged MVEs. Values represent means±s.e.m. ( n ≥48 endosomes; * P <0.001 versus vehicle (open), † P <0.001; Welch’s t -test). Full size image It has recently been shown that ceramide has a role in triggering formation of exosomal ILVs [30] . In view of a causal relationship between S1P signalling and ceramide, the effects of inhibitors of the key enzymes for the generation of ceramide and S1P, that is, sphingomyelinase and SphK, respectively, on CD63 sorting into exosomal ILVs were studied. As compared with a control vehicle, treatment of cells with a neutral sphingomyelinase inhibitor GW4869, which is known to cause a decrease in ceramide content in the cells, caused a strong inhibition of CD63 sorting into exosomal ILVs ( Fig. 5c ), which is consistent with a previous report [30] . This inhibition was rescued by the addition of exogenous cell-permeable C 6 -ceramide. C 6 -ceramide is known to cause enlargement of late endosomes [48] and we confirmed that the short-chain ceramide was well localized at CD63-positive MVEs in HeLa cells ( Supplementary Fig. S10a ). In addition, long-chain ceramide (C 16 -ceramide) also caused a similar effect to C 6 -ceramide ( Supplementary Fig. S10b ). These results may support the importance of ceramide for the generation of ILVs; however, the C 6 -ceramide effect to increase the CD63 sorting into exosomal ILVs was almost completely abrogated by the addition of an SphK inhibitor HACPT. These results suggest that ceramide may not act directly but may act by further being metabolized to S1P. To confirm this notion, the abrogation by HACPT of the C 6 -ceramide effect was cancelled by a photolysis-activated caged S1P but not by an inactive one ( Fig. 5c ). Depletion of S1P signalling decreases exosomal contents For further verification that these CD63-positive ILVs are ipso facto destined for exosome release, exosomes released from the cells were analysed next. Exosomal fractions prepared by a sequential centrifugation from HeLa cells expressing CD63-GFP were examined by an electron microscopy. The final exosome fractions mainly contained small membrane vesicles with a diameter of ~50–100 nm, showing validity of the preparation ( Fig. 6a ). To quantify the amount of CD63 in the exosomes specifically and correctly, the exosomal fractions were first immunoprecipitated with an antibody against an exosomal marker CD81, and the fluorescence corresponding to CD63-GFP in the immunoprecipitated exosomes was measured by a fluorescence-activated cell sorting (FACS) analysis. Importantly, the amount of CD63 in secreted exosomes was reduced in S1P 1 receptor-siRNA or SphK2-siRNA-treated cells ( Fig. 6b ). 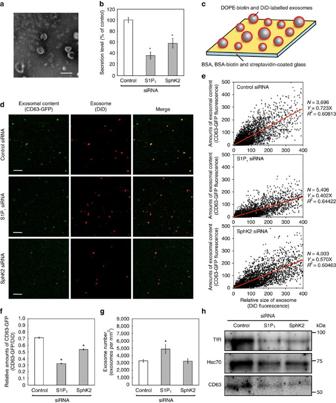Figure 6: Depletion of S1P signalling results in the decrease in exosomal contents. (a) Exosomal fractions prepared by a sequential centrifugation from HeLa cells expressing CD63-GFP were subjected to electron microscopic analysis. Scale bar, 100 nm. (b) The fluorescence intensity corresponding to CD63-GFP in purified exosomal fractions followed by immunoprecipitation by anti-CD81 antibody was quantified by FACS analysis. Values represent means±s.e.m. (n=6; *P<0.001 versus control siRNA (open); Welch’st-test). (c) Biotinylated CD63-GFP-containing exosomes were labelled with a DiD and immobilized on a streptavidin-functionalized surface (see Methods). Images of the two different channels were acquired with a confocal fluorescence microscope. The fluorescence intensities obtained from the images were used to quantify the number of exosomes and relative amounts of CD63-GFP in each exosome. (d) Confocal microscopy images of DiD-labelled exosomes containing CD63-GFP as a cargo tethered on a functionalized glass surface. Scale bars, 10 μm. (e) Correlation diagram between the fluorescence intensity of DiD and that of CD63-GFP in DiD-labelled exosomes (n=3,696, 5,406 and 4,003 exosomes for control, S1P1receptor- and SphK2-siRNA, respectively). (f) The relative amounts of CD63-GFP per DiD fluorescence intensity in each exosome inewere calculated. Values represent means±s.e.m. (*P<0.001 versus control siRNA (open); Welch’st-test). (g) The number of DiD-labelled exosomes indwas quantified. Values represent means±s.e.m. (n=54; *P<0.05 versus control siRNA (open); Welch’st-test). (h) Total exosomal proteins secreted from erythroid-differentiated K562 cells, which had been treated with control, S1P1receptor- or SphK2-siRNA, were analysed by immunoblotting for transferrin receptor (TfR), Hsc70 and CD63. Figure 6: Depletion of S1P signalling results in the decrease in exosomal contents. ( a ) Exosomal fractions prepared by a sequential centrifugation from HeLa cells expressing CD63-GFP were subjected to electron microscopic analysis. Scale bar, 100 nm. ( b ) The fluorescence intensity corresponding to CD63-GFP in purified exosomal fractions followed by immunoprecipitation by anti-CD81 antibody was quantified by FACS analysis. Values represent means±s.e.m. ( n =6; * P <0.001 versus control siRNA (open); Welch’s t -test). ( c ) Biotinylated CD63-GFP-containing exosomes were labelled with a DiD and immobilized on a streptavidin-functionalized surface (see Methods). Images of the two different channels were acquired with a confocal fluorescence microscope. The fluorescence intensities obtained from the images were used to quantify the number of exosomes and relative amounts of CD63-GFP in each exosome. ( d ) Confocal microscopy images of DiD-labelled exosomes containing CD63-GFP as a cargo tethered on a functionalized glass surface. Scale bars, 10 μm. ( e ) Correlation diagram between the fluorescence intensity of DiD and that of CD63-GFP in DiD-labelled exosomes ( n =3,696, 5,406 and 4,003 exosomes for control, S1P 1 receptor- and SphK2-siRNA, respectively). ( f ) The relative amounts of CD63-GFP per DiD fluorescence intensity in each exosome in e were calculated. Values represent means±s.e.m. (* P <0.001 versus control siRNA (open); Welch’s t -test). ( g ) The number of DiD-labelled exosomes in d was quantified. Values represent means±s.e.m. ( n =54; * P <0.05 versus control siRNA (open); Welch’s t -test). ( h ) Total exosomal proteins secreted from erythroid-differentiated K562 cells, which had been treated with control, S1P 1 receptor- or SphK2-siRNA, were analysed by immunoblotting for transferrin receptor (TfR), Hsc70 and CD63. Full size image To get more detailed information on exosomal vesicle maturation, cargo-incorporated exosomes and total exosomes were differentially identified. Purified exosomes were first labelled in a uniform manner with a fluorescent lipophilic tracer (1,1'-dioctadecyl-3,3,3′,3′-tetramethylindodicarbocyanine perchlorate (DiD) dye) and immobilized on a glass surface through streptavidin/biotin affinity ( Fig. 6c ), and the fluorescence intensity of CD63-GFP (cargo-incorporated exosomes) and that of DiD (total exosomes) were quantified simultaneously and analysed ( Fig. 6d,e,f,g ). In a control siRNA-treated cell, the amount of each DiD fluorescence intensity, which reflects the size of exosomes, correlated well with that of CD63, showing well-balanced maturation of exosomal ILVs ( Fig. 6e ). Importantly, when S1P signalling was inhibited by silencing the gene expression of either S1P 1 receptor or SphK2, secreted exosomes showed significantly less amount of CD63 signal without suppressing the DiD signal ( Fig. 6d,e,f ). On the other hand, the total number or size of exosomes was not reduced by silencing the gene expression of either S1P 1 receptor or SphK2 ( Fig. 6d,e,g ). These results, together with the observation that continuous S1P 1 receptor activation is necessary for the cargo sorting into exosomal ILVs, indicate that S1P signalling is indispensable to sorting of cargo molecules into exosomes, while having almost little effects, if any, on ILV formation. As transferrin receptor elimination via exosomes has been accepted for its functional significance during erythrocyte maturation [20] , the effect of S1P signalling on exosome-mediated release of transferrin receptor and related protein Hsc70 was studied. Expectedly, the amounts of transferrin receptor and Hsc70 in secreted exosomes from erythroid-differentiated K562 cells were reduced in S1P 1 receptor-siRNA or SphK2-siRNA-treated cells similar to the result of CD63 ( Fig. 6h and Supplementary Fig. S11 ). Signalling by G protein-coupled receptors is one of the key processes that transmit external signals into cells. In the present studies, we have shown that Gi-coupled S1P receptors on MVEs destined for exosome release undergo ‘ongoing activation’ within the cells through a unique mechanism employing a constant supply of S1P catalysed by SphK2 under resting states. The mechanism underlying how to recruit SphK2 to MVEs has not been clarified yet; however it has been shown that mitogenic signals such as cell activation by serum, which elicits nuclear export of SphK2 by phosphorylation of its nuclear export signal by protein kinase D, thereby resulting in the increase in the cytoplasmic content of SphK2 (refs 49 , 50 ), has a potency to activate S1P 1 receptor on MVEs ( Supplementary Fig. S7 ). As for the activation of catalytic process by the enzyme on MVEs, it may mainly be regulated by its translocation of SphK2 from the cytoplasm to the membrane compartments of MVEs where the substrate sphingosine is enriched [51] , [52] , although direct enzyme activation, such as by phosphorylation [53] , may contribute to some extent. We have also shown that this continuous S1P signalling is indispensable to the cargo sorting into exosomal ILVs. This model will be classified into a unique category of signal transduction: G protein-coupled receptor-mediated signal within organelles. Although the ESCRT machinery is essential for ILV biogenesis in yeast [54] , higher organisms acquired ESCRT-independent mechanisms [55] . The molecular mechanism of regulation in the latter, however, remained unclear. Recently, ceramide was proposed to be a factor involved in ESCRT-independent ILV biogenesis [30] by showing that secreted exosomes purified from oligodendrocyte culture medium are enriched in ceramide, inhibition of neutral sphingomyelinase 2 reduced secretion of exosomes and addition of bacterial sphingomyelinase to liposomes spontaneously induce formation of internal vesicles in vitro . In the present studies, we could partly reproduce their results; for example, sphingomyelinase inhibitor, GW4869, treatment of cells resulted in the inhibition of CD63 sorting into exosomal ILVs of MVEs, whereas the effect of GW4869 was rescued by photolysis-activated caged S1P ( Fig. 5c ). These results indicate that ceramide may be necessary for the ILVs formation but this sphingomyelinase inhibitor treatment also caused effects, through reducing ceramide content, on subsequent metabolite reduction, including S1P, which resulted in a strong inhibition of cargo sorting into exosomal ILVs. As sphingolipid metabolism proceeds rapidly and sequentially, it is attractive to surmise that each metabolite has its own role but has an orchestrated behaviour as a whole, that is, ceramide, having a cone-shaped structure, has a physicodynamic effect on membrane curvature to facilitate inward budding for ILVs formation [56] and a further metabolite S1P has a critical role in the sorting of cargo molecules into ILVs. We have shown that treatment of cells with either SphK inhibitor HACPT or depletion of S1P 1 receptor or SphK2 caused a strong inhibition of CD63 sorting into exosomal ILVs ( Figs 4 and 5 ). It has recently been reported that CD63 directly participates in ESCRT-independent sorting of the Pmel luminal domain into ILVs, and that in the absence of CD63 the Pmel luminal domain is targeted for ESCRT-dependent degradation [29] . It therefore follows that inhibition of CD63 sorting by S1P signalling interference causes a strong suppression of subsequent exosomal cargo sorting. In the ESCRT machinery-dependent ILV formation, these machinery molecules function as a Bin-Amphiphysin-Rvs domain, which can induce and/or sense membrane curvature in the opposite direction. Recently, it has been reported that the βγ subunits of G proteins can also sense membrane curvature [57] . The present studies from our laboratory have demonstrated an ‘ongoing activation’ of Gi-coupled S1P receptors that is necessary for cargo sorting into ILVs destined for exosomal release. It is tempting to speculate that the free βγ subunits that resulted from G-protein activation may be relevant for cargo sorting into ILVs. Another interesting possibility is that S1P signalling has some roles in ILVs formation itself as well. To support this notion, potential roles of G protein subunits in receptor-mediated endocytosis is postulated. Gilman and colleagues [36] have shown that sequestration of heterotrimeric G protein βγ subunits in intact cells strongly inhibits clathrin-coated pit-mediated endocytosis and causes rearrangement of the actin cytoskeleton, and concluded that free βγ subunits of G proteins function to permit endocytosis on activation of G protein-coupled receptors. Another line of evidence suggesting the importance of βγ subunits of G proteins in vesiculation was shown by Malhotra and colleagues [37] , [38] . They have shown that ilimaquinone, a marine sponge metabolite, causes complete vesiculation of the Golgi stacks, and later concluded using an elegantly designed reconstitution assay that ilimaquinone-mediated Golgi vesiculation occurs through activation of heterotrimeric G proteins and that it is the free βγ subunits and not the activated α subunit that triggers Golgi vesiculation. These lines of evidence support a strong link between G protein activation and vesicle formation. To support the importance of Gi protein for vesicular trafficking, recently, an intracellular vesicle-specific splice variant for Gi protein, which regulates vesicular trafficking of dopamine D2 receptors from cellular vesicles to plasma membranes, was identified [58] . Molecular mechanism underlying S1P receptor activation-induced ILV formation in the exosomal MVEs remains to be clarified. The importance of S1P signalling in immunology became clear through a series of studies on an immunosuppressive drug FTY720. It has attracted great attention because of its unique mode of action and its therapeutic interest on immune diseases such as multiple sclerosis. After administration of FTY720, it undergoes phosphorylation by SphK2 and binds with high affinity to S1P receptors and removes them from the cell surface through endocytosis, thereby inducing lymphopoenia [59] . It has been shown that administration of either FTY720 or FTY720-phosphate (FTY720-P) to SJL mice with established relapsing-remitting experimental autoimmune encephalitis resulted in a rapid and sustained improvement in their clinical status; however, the correlation between lymphopoenia and clinical efficacy was imperfect [60] . It means that although the lymphopoenia may be a contributory mechanism to immunosuppression, additional mechanisms may also exist. In this context, we have found that the CD63 sorting into exosomal ILVs was strongly inhibited ( Supplementary Fig. S9a,b ) and that even 6 h after treatment of cells with FTY720-P, S1P 1 receptors were poorly co-localized with CD63-positive MVEs ( Supplementary Fig. S9c ). These results may imply a novel immunosuppressive action of the drug, that is, FTY720 treatment causes inhibition of S1P signalling on MVEs, which blocks exosomal MVE maturation, that may affect early steps of immunization, for example, an exosome-related phenomenon such as antigen presentation by dendritic cells. Indeed, oligodendrocytes secrete relatively large amounts of exosomes enriched in myelin proteolipid protein in the central nervous system, a candidate of autoantigen in multiple sclerosis [30] , [61] . As for the mechanism of depletion of S1P 1 receptors from MVEs, it has recently been shown that S1P 1 receptors were accumulated to Golgi/trans-Golgi network and scarcely found in endosomes for several hours after treatment of cells with FTY720 (ref. 62 ; Supplementary Fig. S9c ). Further studies are necessary to elucidate the immunosuppressive action of the drug. In conclusion, we have demonstrated that in contrast to Gi-coupled S1P receptors in the plasma membrane, those on the CD63-positive exosomal MVEs undergo ‘ongoing activation’ within the organelles. A constant supply of S1P catalysed by SphK2 enables the S1P receptors to be continuously active on the MVEs. Receptor-mediated S1P signalling on MVEs is shown to be essential for cargo sorting into exosomal ILVs. These findings provide a new paradigm for a mechanism underlying ESCRT-independent maturation of exosomal MVEs ( Fig. 7 ). 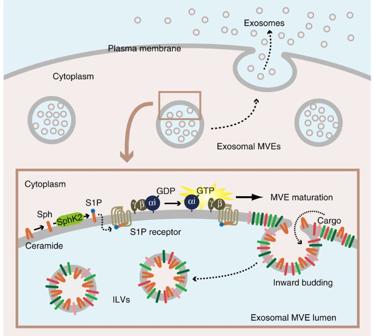Figure 7: Current model for regulation of exosomal MVE maturation by a receptor-mediated S1P signalling. During MVE maturation the lipid composition of ILV membrane dramatically changes, that is, the level of ceramide increases at the expense of sphingomyelin, which is rapidly degraded by various sphingomyelinases65. Ceramide is sequentially metabolized to S1P by SphK2 via sphingosine. On stimulation by S1P, the activation of Gi-coupled S1P receptor triggers the dissociation of Gi subunit Gαi and βγ subunit. This ‘ongoing activation’ of Gi-coupled S1P receptor on the MVE is essential for cargo sorting into exosomal ILVs. Figure 7: Current model for regulation of exosomal MVE maturation by a receptor-mediated S1P signalling. During MVE maturation the lipid composition of ILV membrane dramatically changes, that is, the level of ceramide increases at the expense of sphingomyelin, which is rapidly degraded by various sphingomyelinases [65] . Ceramide is sequentially metabolized to S1P by SphK2 via sphingosine. On stimulation by S1P, the activation of Gi-coupled S1P receptor triggers the dissociation of Gi subunit Gαi and βγ subunit. This ‘ongoing activation’ of Gi-coupled S1P receptor on the MVE is essential for cargo sorting into exosomal ILVs. Full size image Antibodies and reagents The following primary antibodies were used: mouse monoclonal anti-CD63 (clone H5C6, BD); mouse monoclonal anti-EEA1 (clone 14, BD); rabbit polyclonal anti-S1P 1 (H-60, Santa Cruz Biotechnology); mouse monoclonal anti-CD81 (clone JS-81, BD); mouse monoclonal anti-flotillin (clone A-3, Santa Cruz Biotechnology); rabbit polyclonal anti-GM130 (Medical & Biological Laboratories); mouse monoclonal anti-TfR1 (3B8 2A1, HyCult Biotech); rat monoclonal anti-Hsc70 (1B5, Stressgen Biotech); mouse monoclonal anti-α tubulin (B-5-1-2, Sigma-Aldrich). A rabbit polyclonal antibody against the amino terminus of SphK2 (anti-SphK2) has been described previously [49] . Alexa-Fluor secondary antibodies were obtained from Life Technologies. Horseradish peroxidase (HRP)-conjugated goat anti-mouse IgG antibody and HRP-conjugated goat anti-rabbit IgG antibody were purchased from Bio-Rad. HRP-conjugated goat anti-rat IgG antibody was purchased from Jackson ImmunoResearch. S1P and C 16 -ceramide were purchased from Enzo Life Sciences. Caged S1P and FTY720-phosphate were purchased from Santa Cruz Biotechnology. ADP, W146, nocodazole, GW4869, C 6 -ceramide and BSA-biotin were purchased from Sigma-Aldrich. Alexa647-EGF and BODIPY TR-C 5 -ceramide were purchased from Life Technologies. HACPT was purchased from Calbiochem. PTX was purchased from Wako Pure Chemical Industries. JTE-013, BML-241 and FTY720 (fingolimod) were purchased from Cayman Chemical. 1,2-Dioleoyl-sn-glycero-3-phosphoethanolamine-N-(cap biotinyl) (sodium salt) (DOPE-biotin) was purchased from Avanti. Streptavidin and DiD were purchased from Molecular Probes. Hemin was purchased from Alfa Aesar. All other materials were reagent grade. Plasmids and mutations Human SphK2-GFP and murine S1P 1 -CFP were constructed as described previously [41] , [50] . Murine S1P 3 was amplified and cloned into pECFP-N1 (Clontech) and pEGFP-N1 (Clontech) for making CFP- or GFP-tagged S1P 3 , respectively. Human S1P 2 was amplified and cloned into pEGFP-N1 (Clontech) for making GFP-tagged S1P 2 . Murine S1P 1 from the S1P 1 -CFP was subcloned into pEYFP-N1 (Clontech) for making YFP-tagged S1P 1 . Human Gαi and human Gβ1were amplified and cloned into pECFP-N1 (Clontech) for making CFP-tagged Gαi or intact Gβ1. Human Gγ2 was amplified and cloned into pEYFP-N1 (Clontech) for making YFP-tagged Gγ2. Human CD63 was amplified and cloned into pEGFP-N1 or pmCherry-N1 (Clontech) for making GFP- or mCherry-tagged CD63, respectively. Human Rab5 was amplified and cloned into FLAG-pCMV5 for making N-terminally FLAG-tagged Rab5. For FLAG-Rab5 (Q79L), glutamine 79 was mutated to a leucine using a QuickChange site-directed mutagenesis protocol. DsRed-tagged Rab5 (Q79L) was generated by subcloning the Rab5 (Q79L) into pDsRed-monomer-C1 (Clontech). For PCR amplification, we used the primers (Hokkaido System Science) as listed in Supplementary Table S1 . Short interfering RNAs For RNA interference, we used the oligonucleotides (Japan Bio Services, Saitama, Japan) as described previously [30] , [63] and listed in Supplementary Table S2 . Cell cultures and transfections HeLa cells purchased from Riken Cell Bank (Tsukuba, Japan) were maintained in DMEM medium (Wako Pure Chemical Industries) containing 10% fetal bovine serum and 1% penicillin/streptomycin at 37 °C in 5% CO 2 . HUVEC were purchased from PromoCell and maintained in endothelial cell growth medium containing endothelial cell growth supplement (PromoCell). HUVEC between passages 2 and 5 were used in the experiments described herein. K562 cells purchased from Riken Cell Bank were maintained in RPMI1640 medium (Wako Pure Chemical Industries) containing 10% fetal bovine serum and 1% penicillin/streptomycin at 37 °C in 5% CO 2 . Cells were plated onto glass-bottomed 35 mm culture dishes (MatTek) before transfection. Transient transfection was carried out using FuGENE HD (Promega) for HeLa cells or Lipofectamine 2000 (Life Technologies) for HUVEC. In the case of siRNA experiments, transient transfection was carried out using Lipofectamine 2000 for HeLa cells or HUVEC and Lipofectamine RNAiMAX (Life Technologies) for K562 cells. All experiments were performed 2 to 3 days after transfection. For erythroid differentiation, K562 cells were seeded at a density of 8 × 10 5 cells per ml and cultured for 24 h in the presence of 10 μM hemin. Loading of caged S1P HeLa cells grown on glass-bottomed culture dishes were preloaded with 1 μM caged S1P for 30 min. After washing out the media, dishes were then flashed with ultraviolet light (254 nm) for 20 s for photolysis of caged S1P. Next, cells were incubated in culture condition for indicated time. Immunocytochemistry HeLa cells were fixed with a fixative containing 4% paraformaldehyde in PBS (pH 7.4) for 15 min. After washing twice with PBS, cells were treated with PBS containing 0.3% Triton X-100 for 3 min, then 10% normal goat serum for 10 min. Cells were then incubated with the anti-CD63 monoclonal antibody (diluted 1:200), anti-EEA1 monoclonal antibody (diluted 1:200), anti-S1P 1 polyclonal antibody (diluted 1:2,000), anti-SphK2 polyclonal antibody (diluted 1:2,000), anti-CD81 monoclonal antibody (diluted 1:200), anti-flotillin monoclonal antibody (diluted 1:200) or anti-GM130 polyclonal antibody (diluted 1:200) in PBS for 24 h at 4 °C. After washing in PBS, cells were incubated with Alexa-Fluor 488, Alexa-Fluor 594 goat anti-mouse or anti-rabbit IgG (diluted 1:1,000) for 30 min. After washing three times with PBS for 10 min each, the fluorescence was observed under a confocal laser scanning microscope (LSM 510 META, Carl Zeiss) using a × 63 oil plan-apochromat objective (numerical aperture, 1.4; Carl Zeiss), with excitation at 458 nm using a 475–525-nm band-pass barrier filter for CFP, with excitation at 488 nm using a 505–530-nm band-pass barrier filter for GFP and Alexa488, with excitation at 543 nm using a 560-nm long-pass barrier filter for mCherry and Alexa594, and with excitation at 633 nm using a 650-nm long-pass barrier filter for Alexa647. FRET analysis HeLa cells were transiently cotransfected with Gαi-CFP (donor), Gβ and Gγ-YFP (acceptor), or S1P 1 -CFP (donor), Gβ and Gγ-YFP (acceptor) at a donor/acceptor ratio of 1:1. Three days after cotransfection, cells were fixed and each area of interest was subjected to FRET analysis with acceptor photobleaching method using a LSM 510 META with a × 63 oil plan-apochromat objective. Following excitation at 458 or 514 nm, CFP emission with a 475–525-nm band-pass barrier filter or YFP emission with 530–600-nm band-pass barrier filter, respectively, was collected. In the case of codetection of mCherry fluorescence, following excitation at 543 nm, mCherry emission with a 650-nm long-pass barrier filter was collected. An area of interest was selected for photobleaching of YFP. A protocol was then used, which recorded pre- and post-bleaching images using 458 nm excitation at 10% laser power to limit photobleaching, with a bleaching of the selected area with 100%, 514 nm laser power for 100 of iteration (acceptor photobleaching). FRET was resolved as an increase in the CFP (donor) signal after photobleaching of YFP (acceptor). FRET efficiency ( E ) can be determined from the relative fluorescence intensity of the energy donor (CFP) before ( I pre ) and after ( I post ) photobleaching of the energy acceptor (YFP): E =1−( I pre / I post ). FRAP analysis FRAP analysis was performed using LSM 510 META with a × 63 oil plan-apochromat objective as described previously [41] . Briefly, HeLa cells expressing SphK2-GFP and CD63-mCherry were pretreated with 10 μM nocodazole in Hanks’ balanced salt solution (HBSS, Sigma Aldrich) containing 1 mM CaCl 2 and 5 mM HEPES buffer for 30 min. SphK2-GFP fluorescence was monitored with excitation at 488 nm using a 505–530-nm band-pass barrier filter. Each square region of a CD63-mCherry-positive vesicle or cytoplasm of interest was photobleached by scanning with 100%, 488 nm laser at the highest power. Recovery of fluorescence in the selected regions was then analysed with low laser power at the indicated times after photobleaching. For all of the images, noise levels were reduced by line scan averaging. Analysis of cargo sorting into MVEs HeLa cells expressing CD63-GFP and Rab5 (Q79L)-DsRed, or HeLa cells expressing CD63-GFP and FLAG-Rab5 (Q79L) were fixed 3 days after transfection. Images were then obtained using a LSM 510 META with a × 63 oil plan-apochromat objective, optical zooms with × 6 and optical slice <0.9 μm. The amount of CD63-GFP in the endosomal lumen was quantified as fluorescence intensity in the lumen versus the limiting membrane of enlarged vesicle (diameter; >1 μm). In some experiments, endogenous CD81 and flotillin were immunostained with anti-CD81 or anti-flotillin antibodies (secondary antibody; Alexa-Fluor594 goat anti-mouse IgG) as described in ‘Immunocytochemistry’. The amount of CD63-GFP, CD81 or flotillin in the endosomal lumen was quantified as fluorescence intensity in the lumen versus the limiting membrane of enlarged vesicle (diameter >1 μm). For simultaneous observation of CD63-GFP and Alexa647-EGF, HeLa cells expressing CD63-GFP and Rab5 (Q79L)-DsRed for 3 days were treated with 100 ng ml −1 Alexa647-EGF for 30 min and fixed. Images were then obtained and quantified as described above. Live-cell imaging of cargo sorting into MVEs HeLa cells expressing CD63-GFP and Rab5 (Q79L)-DsRed were loaded for 30 min with 1 μM caged S1P in cultured condition, followed by rinsing with HBSS. Cells were then pretreated with 10 μM nocodazole with or without 5 μM HACPT in HBSS containing 1 mM CaCl 2 and 5 mM HEPES for 30 min. In some experiments, cells were pretreated with 100 ng ml −1 PTX for 3 h before the nocodazole treatment. CD63-GFP fluorescence was monitored using a LSM 510 META with a × 63 oil plan-apochromat objective at 37 °C. Next, each lumen of enlarged vesicle was photobleached by scanning with a 488-nm wavelength of argon laser at the highest power. Recovery of fluorescence in the lumen was then analysed with low laser power after photobleaching. Five minutes after the photobleaching, the whole region of the inside of the cells was then scanned with a 351-nm wavelength of ultraviolet laser at the highest power for photolysis of caged S1P. Images were then obtained with low laser power of 488 nm after photolysis. Exosome purification HeLa cells were transfected with CD63-GFP and indicated siRNAs. Forty-eight hours after the transfection, medium was changed to ‘exosome-depleted medium’, where exosomes in culture medium were removed by overnight centrifugation at 100,000 g (ref. 64 ) and cells were cultured for 24 h. Cell culture media were collected and centrifuged for 10 min at 500 g and for 20 min at 12,000 g , then supernatants were purified by filtration on 0.22 μm pore filters, followed by ultracentrifugation for 70 min at 100,000 g . The fractions were then resuspended in PBS–1% BSA. Electron microscopy HeLa cells expressing CD63-GFP were transfected with control siRNA, exosomes were prepared, fixed with 4% paraformaldehyde and 4% glutaraldehyde, washed in PBS, negatively stained with 2% phosphotungstic acid and viewed using a JEM-1200EX transmission electron microscope (JEOL) at 80 kV. Immunoadsorption and detection of exosomes by FACS Anti-CD81 antibody was coupled to 4 μm aldehyde-sulphate beads (Life Technologies) by incubating 7 μg of antibody with 2 × 10 7 beads. Cleared supernatants of purified exosome fraction were incubated with 20,000 of anti-CD81-coupled beads overnight at room temperature. After washing, beads were acquired on a FACSCalibur (BD) [64] . Quantification of content and size of each exosome Exosomal content quantification assay was performed by fluorescence-based single liposome assay [57] . HeLa cells were seeded at 5 × 10 5 cells on 60 mm culture dish and cells were transfected with CD63-GFP and indicated siRNAs. Forty-eight hours after the transfection, medium was changed to ‘exosome-depleted medium’ and cells were cultured for 24 h. One-third of the purified exosomes were incubated with a mixture of 100 mg l −1 DOPE-biotin and 10 mg l −1 DiD for 10 min. Glass coverslip in glass-bottomed 35 mm culture dish (MatTek) was incubated with a mixture of 0.1 g l −1 BSA/BSA–biotin, 10:1, in distilled water for 10 min. Excess protein was removed by gently flushing the surface with PBS and subsequently incubated for 10 min with 0.025 g l −1 streptavidin. The surface was gently rinsed with PBS. DOPE-biotin- and DiD-labelled exosomes were added onto the surface-functionalized glass coverslip and incubated for 30 min. The surface was gently rinsed with PBS. The fluorescence of GFP and DiD are observed under a confocal laser scanning microscope (LSM 510 META) using a × 63 oil plan-apochromat objective, with excitation at 488 nm using a 505–530-nm band-pass barrier filter for GFP, with excitation at 633 nm using a 650-nm long-pass barrier filter for DiD. Cell surface protein labelling and isolation HeLa cells transfected with S1P 1 -CFP were treated with 100 nM S1P and then cell surface proteins were biotinylated using Cell Surface Protein Isolation Kit (Pierce) with Sulpho-NHS-SS-Biotin according to the manufacturer’s instructions. Biotinylated cell surface proteins were isolated using an immobilized NeutrAvidin Gel and subjected to immunoblotting. Immunoblotting The purified exosomes derived from the erythroid differentiated K562 cells were detergent-solubilized and separated on 10–12% SDS–PAGE gels, blotted polyvinylidene difluoride membrane (Millipore), probed with the anti-TfR1 monoclonal antibody (diluted 1:50), anti-Hsc70 monoclonal antibody (diluted 1:1,000) or anti-CD63 monoclonal antibody (diluted 1:1,000). HRP-conjugated secondary antibodies were revealed using SuperSignal West Dura Extended Duration Substrate (Thermo Fisher Scientific). Images were acquired using LAS1000 (Fujifilm). After solubilization, the biotinylated cell surface proteins were collected with immobilized NeutrAvidin Gel, separated by 10% SDS–PAGE gels followed by immunoblotting with the anti-S1P 1 polyclonal antibody (diluted 1:1,000) or anti-α tubulin monoclonal antibody (diluted 1:5,000), visualized with HRP-conjugated secondary antibody using SuperSignal West Dura Extended Duration Substrate and analysed by LAS1000 or LAS3000 (Fujifilm). Full-length images of immunoblottings are shown in Supplementary Fig. S11 . Statistical analyses Results are expressed as means±s.e.m. Data were analysed by Welch’s t -test using the MedCalc statistical software (MedCalc Software). P- values <0.05 were considered significant. Error bars indicate s.e.m. How to cite this article: Kajimoto, T. et al. Ongoing activation of sphingosine 1-phosphate receptors mediates maturation of exosomal multivesicular endosomes. Nat. Commun. 4:2712 doi: 10.1038/ncomms3712 (2013).